Towards a general diastereoselective route to oxabicyclo[3.2.1]octanes via a gold-catalysed cascade reaction The development of an efficient diastereoselective synthesis of the oxabicyclo[3.2.1]octane ring system bearing two oxygenated quaternary chiral centres represents a significant challenge. This motif can be found in a wide range of natural products with significant biological activities. Here we report the synthesis of such kind of scaffold using a cyclohexane- trans -1,4-diol with an alkyne side chain in the presence of Au(I) catalyst. This is a domino process in which two C–H, two C–O and one C–C bond is assembled through a sequence of cyclization/semi-pinacol rearrangements. This strategy has been successfully applied to the asymmetric formal total synthesis of (+)-cortistatins. A wide variety of intriguing natural products with 8-oxabicyclo[3.2.1]octane motifs ( 1 – 8 , Fig. 1 ) have been shown to exhibit significant biological activities. 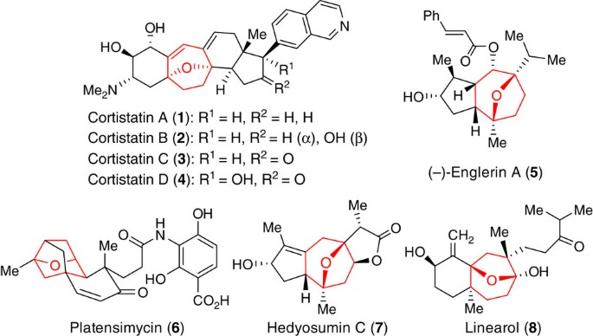Figure 1: Representative natural products containing oxa-bridged seven-membered carbocycles. Selected biologically active natural products bearing functionalized 8-oxabicyclo[3.2.1]octane rings. Figure 1: Representative natural products containing oxa-bridged seven-membered carbocycles. Selected biologically active natural products bearing functionalized 8-oxabicyclo[3.2.1]octane rings. Full size image The cortistatins ( 1 – 4 ) are a family of 11 steroidal alkaloids, with unique structures and prominent biological activities [1] , [2] . They were isolated from the marine sponge Corticium simplex by the Kobayashi group in 2006 and 2007. Among them, cortistatin A ( 1 ) has proved to be the strongest inhibitor of the migration and proliferation of human umbilical vein endothelial cells at concentrations as low as 100 pM, and with a therapeutic index of over 3,300. Englerin A ( 5 ) is isolated from the stem bark of Phyllanthus engleri in Tanzania. It is a guaiane sesquiterpene and has been reported to selectively inhibit the growth of renal cancer cell lines at the nanomolar level [3] . Platensimycin ( 6 ) comes from the fermentation broth of Streptomyces platensis . It is a broad-spectrum antibiotic against Gram-positive bacteria and exerts its antibacterial effect by selectively inhibiting the β-ketoacyl-(acyl-carrier-protein)synthase (FabF), one of the key enzymes in bacterial fatty acid biosynthesis [4] , [5] . Hedyosumin C ( 7 ), isolated from Hedyosmum orientale , represents a novel type of sesquiterpenoid with cytotoxic activity against human lung adenocarcinoma and leukaemia tumour cell lines [6] . Linearol ( 8 ), isolated from dried Dictyota Indica , has a significant inhibitory effect on herbivores [7] . The biological properties, together with their complex structures have elevated them to be prominent targets for total synthesis [8] , [9] , [10] , [11] , [12] , [13] . However, the challenges associated with the diastereoselective synthesis of the 8-oxabicyclo[3.2.1]octane core reside in construction of the two oxygenic quaternary chiral centres. A general diastereoselective route for the development of divergent synthetic processes to produce assortments of skeletally diverse and densely functionalized oxabicyclo[3.2.1]octane scaffolds is always highly desirable, despite the excellent progress made thus far [14] , [15] , [16] , [17] , [18] , [19] , [20] , [21] , [22] , [23] , [24] . Herein we report a general strategy using a semi-pinacol rearrangement cascade reaction of substituted 1-ethynylcyclohexane- trans -1,4-diols. This goes via a highly strained oxonium ion generated in situ and is derived from nucleophilic addition of a hydroxyl group onto a gold-activated alkyne. This chemistry has been successfully applied to the asymmetric formal total synthesis of (+)-cortistatins. The cascade reaction [25] allows several bond-forming and/or -cleaving events to occur in a single synthetic operation, thus minimizing the costs and waste. Over the past 10 years, gold catalysts have risen to the forefront of cycloisomerization due to their high activities and the mild reaction conditions, and a wide variety of organic scaffolds are available by these methods [26] , [27] , [28] , [29] . As a soft Lewis-acid catalyst, gold complex could selectively activate alkynes and promote the addition of nucleophiles [30] . In this context, the intramolecular nucleophilic addition of a hydroxyl group to a Au-activated carbon–carbon triple bond, followed by a compatible synthetic transformation has proven to be a powerful method for the synthesis of structurally diverse scaffolds ( Fig. 2a ) [31] , [32] , [33] . 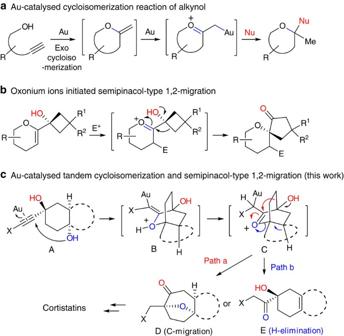Figure 2: Gold-catalysed sequential reactions. (a) Au-catalysed cycloisomerization of alkynol to generate structurally diverse oxacycles; (b) semi-pinacol-type 1,2-migration of oxonium ions to construct oxaspirocycles; (c) our strategy to access oxabicyclo[3.2.1]octane ring systems via Au-catalysed annulations and the application to cortistatins synthesis. Figure 2: Gold-catalysed sequential reactions. ( a ) Au-catalysed cycloisomerization of alkynol to generate structurally diverse oxacycles; ( b ) semi-pinacol-type 1,2-migration of oxonium ions to construct oxaspirocycles; ( c ) our strategy to access oxabicyclo[3.2.1]octane ring systems via Au-catalysed annulations and the application to cortistatins synthesis. Full size image On the other hand, 1,2-alkyl migration has been considered as a key element in numbers of novel gold-catalysed cascade reactions [34] , and it could be induced through oxonium ions [35] , [36] or gold carbenoids [37] , [38] , [39] , [40] . Recently, the electrophile-induced intermolecular addition of enol ether, followed by semi-pinacol-type 1,2-migration of the resulting oxonium ions has been well documented to be a powerful method to synthesize several complex natural products by Tu and colleagues [41] ( Fig. 2b ). In accordance with our goal, an oxygenated quaternary chiral center was generated from the corresponding hydroxyl vinyl ether. On the basis of previous work in our laboratory using gold-catalysed tandem reactions of alkynes with internal nucleophiles [42] , [43] , we wondered if oxabicyclo[3.2.1]octane scaffolds D could be constructed from 1-ethynyl-cyclohexane- trans -1,4-diol A via a gold-catalysed cascade reaction ( Fig. 2c ). Formation of the tricyclic oxabicyclo[3.2.1]octane scaffold D was envisioned to come about from an intramolecular 6-exo-dig nucleophilic addition of the OH group in substrate A onto the Au-activated triple bond, and the resultant exo-cyclic enol ether B was expected to undergo an isomerization to the highly strained oxonium ion C , followed by a semi-pinacol-type 1,2-alkyl migration (path a) to give the oxabicyclo[3.2.1]octane scaffold D , or via a β-hydrogen elimination (path b) to the bicyclic product E . Whilst this proposed cascade reaction is unknown, there have been reports of Au-catalysed nucleophilic addition of hydroxyl groups to alkynes [44] , Au-catalysed isomerization of an exo-cyclic enol ether [45] , [46] and the oxonium-induced semi-pinacol rearrangement [34] , [41] . Optimization of reaction conditions Model substrates were first used to test the feasibility of the proposed strategy outlined in Fig. 2 ( Table 1 ). To this end, 1-ethynyldecahydro-naphthalene-1,4-diol 9 was treated with AuCl and AuCl 3 in 1,2-dichloroethane at room temperature. This gave the desired 8-oxabicyclo[3.2.1]octane 10 in 69% and 48%, respectively (entries 1 and 2; Table 1 ). Tests revealed Ph 3 PAuNTf 2 (5 mol%) to be the optimum gold catalyst when used at room temperature for 2 h and gave 10 in 72% yield (entries 3–6; Table 1 ). In terms of solvent, dichloromethane (DCM) gave better results than dichloroethane and toluene (entries 7 and 8). Decreasing the loading of Ph 3 PAuNTf 2 had little effect on the yield (entry 9). Platinum catalysts can also be used for alkyne-based hydroelement addition reactions. However, in this case only starting material was recovered when K 2 PtCl 6 was used and for PtCl 2 a yield of only 28% was observed (entries 10 and 11). Alternative Lewis acid or Brønsted acid, such as N -iodosuccinimide or p -toluenesulfonamide had no effect on the reaction, however substrate decomposition was observed when the reaction time was extended or the temperature increased (entries 12 and 13). A control experiment in the absence of gold catalyst gave no desired product, indicating that Ph 3 PAuNTf 2 is essential (entry 14). In light of these results, the optimized conditions for this reaction are Ph 3 PAuNTf 2 (2.5 mol%) in DCM at room temperature. The experimental conditions were particularly practical because neither flame-dried glassware, an inert atmosphere nor carefully dried solvent were required. Table 1 Sequential reaction of diol 9 with various catalysts*. Full size table Substrate scope A number of substituted 1-ethynyldecahydronaphthalene-1,4-diols ( Table 2 ) were used to assess the generality of this reaction. These substrates bearing electron-withdrawing groups, such as bromide, iodide and ester on the terminal alkyne were synthesized ( 11a – 11c ). The corresponding products 12a – 12c were obtained in good yields, allowing the further functional group inter-conversion to facilitate the synthetic transformation (entries 1–3). In addition, when the terminal alkynes had phenyl, allyl or alkyl substituents ( 11d – 11f ), the expected annulated products ( 12d – 12f ) were formed albeit in slightly lower yields (entries 4–6). Notably, when the alkyne moiety had an alkyl group, hydrogen elimination was a potential competing reaction and gave 13f in 21% yield (entry 6). Table 2 Au-catalysed sequential reactions with alkyne-substituted bicyclic diols*. Full size table Methoxyethoxymethyl (MEM) protection of the hydroxyl group at C4 led to product 12g in 65% yield, indicating the reaction might proceed via the intramolecular nucleophilic addition of the MEM ether to the Au-activated alkyne, followed by deprotection of the MEM group (entry 7). Furthermore, the [6,5]-fused bicyclic substrates also underwent the sequential reaction to give the desired products in excellent yields (entries 8–11). The relative stereochemistry of 12k was confirmed by X-ray crystallography. The bulky alkyl group and electronic effect of the ester in substrates 11c , 11f and 11k meant that the reaction had to be carried out at higher temperature (70 °C) to accelerate the addition of the tertiary hydroxyl group to the triple bond. It is worthwhile to mention that when substrate 11l was used, 14 was obtained in 85% yield. This supports our proposed formation of intermediate B ( Fig. 2c ). Interestingly, further treatment of 14 with gold catalyst at high temperature (70 °C) afforded 15 in 91% yield, presumably through intermediate 13l ( Fig. 3 ). Alternative acids, such as TsOH, HCl, AcOH, AlCl 3 and AlMe 3 , all failed to promote this transformation. 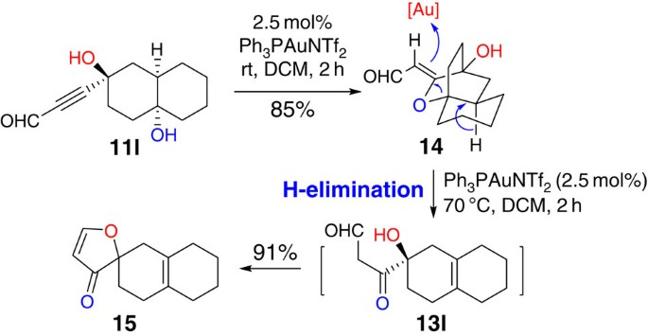Figure 3: H-elimination pathway for the propargyl aldehyde substrate. A cyclization intermediate14could be isolated from the Au-catalysed reaction of propargyl aldehyde substrate11l. Further treatment with gold catalyst in higher temperature,14could undergo H-elimination, followed by a condensation to afford spiro-compound15. Figure 3: H-elimination pathway for the propargyl aldehyde substrate. A cyclization intermediate 14 could be isolated from the Au-catalysed reaction of propargyl aldehyde substrate 11l . Further treatment with gold catalyst in higher temperature, 14 could undergo H-elimination, followed by a condensation to afford spiro-compound 15 . Full size image The Au-catalysed sequential reaction of monocyclic diol substrates were also tested ( Table 3 ) for the synthesis of 8-oxabicyclo[3.2.1]octane derivatives equipped with several functional groups. These are useful in the synthesis of natural products containing this basic skeleton, such as (−)-englerin A ( 5 ), platensimycin ( 6 ), hedyosumin C ( 7 ) and linearol ( 8 ), and also for the preparation of a variety of valuable functionalized cyclic compounds. Table 3 Au-catalysed sequential reactions of alkyne-substituted monocyclic diols*. Full size table The reaction of substrates 16a – 16h generated desired products 17a – 17h in good yields ( Table 3 ). Substrates bearing a terminal alkyne and those substituted with halogen atoms or an ester tolerated the reaction conditions. These groups allow further functional group manipulation (entries 1–4; Table 3 ). R group has proven to be compatible with a variety of functional groups, such as alkyl group, allyl group or even just H atom (entries 5–8). In the case where R=H (entry 8), a higher temperature was required. This may be because the distance between the secondary hydroxyl group and the alkyne is greater than that in the case of tertiary alcohol-based substrates. Mechanistic investigation In our proposed mechanism for this Au-catalysed cascade reaction ( Fig. 4 ), the alkyne moiety of the substrate is first activated by the active catalyst Ph 3 PAuNTf 2 , which is generated from the reaction between Ph 3 PAuCl and AgNTf 2 (ref. 47 ), to form π -coordinated intermediate A . The subsequent intramolecular nucleophilic attack by the hydroxyl group takes place to form a [2.2.2] bicyclic intermediate B , which would isomerize to a highly strained oxonium intermediate C through a proton shift [48] . Oxonium ion-initiated semi-pinacol rearrangement could afford intermediate D or E through pathway 1 or 2 and release ring strain. The following proton shift would form product 10 or side product 10′ , respectively, and regenerate the active catalyst Ph 3 PAuNTf 2 (ref. 49 ). 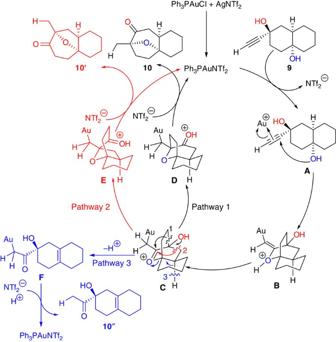Figure 4: Proposed mechanism for the Au-catalysed annulation reaction. The proposed mechanism involves the sequential intramolecular nucleophilic addition/ 1,3-proton shift/ oxonium ion-initiated semi-pinacol rearrangement (pathways 1 and 2) or hydrogen elimination (pathway 3). Figure 4: Proposed mechanism for the Au-catalysed annulation reaction. The proposed mechanism involves the sequential intramolecular nucleophilic addition/ 1,3-proton shift/ oxonium ion-initiated semi-pinacol rearrangement (pathways 1 and 2) or hydrogen elimination (pathway 3). Full size image Alternatively, H-elimination followed by C–O bond cleavage would form intermediate F , which could lead to the generation of another side product 10′′ (pathway 3) [50] . Although path 3 was observed in some cases (for substrate 11f and 11l ), path 2 was never detected. To gain further insights into the mechanism and the origins of the excellent regioselectivity of the semi-pinacol type of 1,2-alkyl migration, we completed detailed density functional theory (DFT) calculations. Computational study The M11-L/6-311+G(d)//B3LYP/6-31+G(d) (Stuttgart/Dresden effective core potentials (SDD) basis set for Au atom) calculated free-energy profiles for the Au-catalysed annulation reaction are shown in Fig. 5a to clarify the mechanisms proposed in Fig. 4 . All of the DFT calculations conducted in this study were carried out using the GAUSSIAN 09 series of programs [51] . DFT method B3LYP (refs 52 , 53 ) with a standard 6-31+G(d) basis set (SDD basis set for Au) was used for the geometry optimizations. The M11-L functional, proposed by Peverati and Truhlar [54] , was used with a 6-311+G(d) basis set (SDD basis set for Au) to calculate the single point energies. The solvent effects were taken into consideration using single point calculations based on the gas-phase stationary points with a SMD continuum solvation model [55] , [56] , [57] . The energies presented in this paper are the M11-L calculated Gibbs free energies in a DCM solvent with B3LYP calculated thermodynamic corrections. 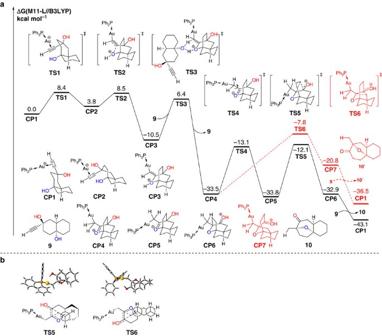Figure 5: Free-energy profiles for the two competing mechanisms. (a) SMD-M11-L/6-311+G(d)//B3LYP/6-31+G(d) (SDD for Au) calculated free-energy profile for the sequence of intramolecular nucleophilic addition/semi-pinacol rearrangement of 1-ethynylcyclohexane-trans-1,4-diols established in this study for the reaction of key intermediateCP1. This indicates that the semi-pinacol rearrangement is the rate-determining step of this reaction and formation of complex10via transition stateTS5is both thermodynamically and kinetically favourable (seeSupplementary Tables 1 and 2). (b) The Newman projections of transition states TS5 and TS6. Figure 5: Free-energy profiles for the two competing mechanisms. ( a ) SMD-M11-L/6-311+G(d)//B3LYP/6-31+G(d) (SDD for Au) calculated free-energy profile for the sequence of intramolecular nucleophilic addition/semi-pinacol rearrangement of 1-ethynylcyclohexane- trans -1,4-diols established in this study for the reaction of key intermediate CP1 . This indicates that the semi-pinacol rearrangement is the rate-determining step of this reaction and formation of complex 10 via transition state TS5 is both thermodynamically and kinetically favourable (see Supplementary Tables 1 and 2 ). ( b ) The Newman projections of transition states TS5 and TS6. Full size image Initially, the alkynediol-coordinated Au-complex CP1 was set to the relative zero of the relative free energy. The ring flip, which gives intermediate CP2 with boat conformation, occurs via a twisted boat transition state TS1 with a barrier of 8.4 kcal mol −1 . The Au-activated alkynediol CP2 might undergo an intramolecular nucleophilic addition of its hydroxyl group to the triple bond in an exo-selective manner to give oxinum ionic intermediate CP3 , via transition state TS2 with an energetic span of 4.7 kcal mol −1 . The intermolecular hydrogen shift between intermediate CP3 and 9 (or water [58] ) irreversibly gives carbocation intermediate CP4 , via transition state TS3 with an energetic span of 16.9 kcal mol −1 . Subsequently, the conformational isomerization of CP4 gives carbocation intermediate CP5 , via transition state TS4 with a barrier of 20.4 kcal mol −1 . The carbocation intermediate CP5 undergoes a semi-pinacol rearrangement via transition state TS5 with a barrier of 21.7 kcal mol −1 to give intermediate CP6 . The following proton shift and coordination of 9 gives the major product 10 with 31.0 kcal mol −1 exothermic. Alternatively, side product 10′ would also be formed by the semi-pinacol rearrangement of another carbon atom via transition state TS6 from CP4 . The relative free energy of transition state TS6 is 4.3 kcal mol −1 higher than that of transition state TS5 . Therefore, complex 10′ cannot be observed experimentally. This result is consistent with the experimental observation. The Newman projections of transition states TS5 and TS6 are shown in Fig. 5b to further demonstrate the regioselectivity of the semi-pinacol rearrangement, in which the axis in the projections is supposed to rotate accordingly along with the migration. In transition state TS5 , when the carbon atom migrates, the axis of Newman projection, being located out of the cyclohexane ring, rotates anticlockwise without restriction. In transition state TS6 , however, the cyclohexane ring restricts the free rotation of the axis on it in Newman projection. Hence, the strain coming from the conformational change of the cyclohexane ring in transition state TS6 blocks the carbocation rearrangement. Formal synthesis of the cortistatins The high yields and mild reaction conditions make this reaction to be a desirable method to construct oxabicyclo[3.2.1]octane scaffolds. These are present in the cortistatins and inspired us to attempt their total synthesis [59] , [60] , [61] , [62] , [63] , [64] , [65] , [66] , [67] . Our retrosynthetic analysis of cortistatins A , L , J and K is shown in Fig. 6 . Inspiration came from the highly efficient synthesis of cortistatins from tetracyclic intermediate 18 reported by Myers and colleagues [65] . Ketone 19 (Br being a substituent capable of S N 2 displacement) could be a precursor to intermediate 18 , and it might be synthesized by our gold-catalysed cascade reaction from alcohol 20 , which in turn could be made from ketone 21 via an alkynation. This ketone could be derived from Hajos–Parrish ketone 22 . 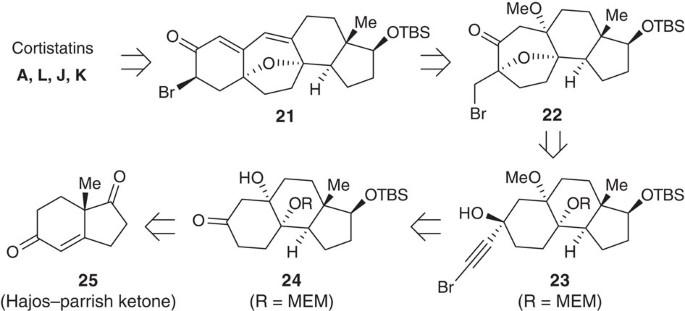Figure 6: Retrosynthetic analysis of cortistatins. The current Au-catalysed annulation reaction was used as a key step to construct the oxabicyclo[3.2.1]octane ring. Figure 6: Retrosynthetic analysis of cortistatins. The current Au-catalysed annulation reaction was used as a key step to construct the oxabicyclo[3.2.1]octane ring. Full size image Our synthesis commenced with known compound 21 ( Fig. 7 ), which was prepared from Hajos–Parrish ketone 22 by a modified procedure reported by Shair and colleagues [63] (see Supplementary Methods ). Initial attempts to protect the tertiary alcohol as the methyl ether were unsuccessful. Decomposition was observed presumably because of the ketone at the β-position of the tertiary hydroxyl group. A stepwise approach was adopted, whereby 21 was first treated with Pyridinium p-Toluenesulfonate (PPTS) in the presence of 2,2-dimethylpropane-1,3-diol and the resultant ketal was then protected as its methyl ether using MeI/KH in tetrahydrofuran (THF). Removal of the ketal group [68] gave 23 in 40% yield over the three steps. 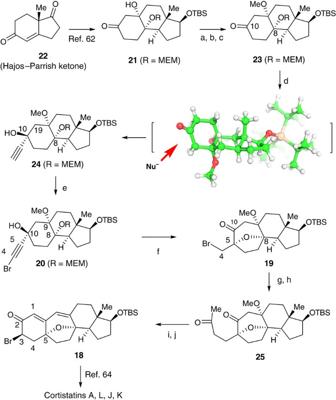Figure 7: Formal total synthesis of the cortistatins. (a) 2,2-Dimethylpropane-1,3-diol, Pyridinium p-Toluenesulfonate (PPTS) benzene, 50 °C, 4 h, 80%; (b) KH, MeI, THF, 0 °C to room temperature (rt), 92%; (c) CAN, borate buffer (pH=8.0), 60 °C, 5 h, 55%; (d) ethynylmagnesium chloride, THF, 0 °C to rt, 75%+20% diastereomer; (e) NBS, AgNO3, acetone, rt, 0.5 h, 90%; (f) Ph3PAuNTf2(2.5 mol%), DCM, rt, 1 h, 81%; (g) allyl(Bu)3Sn, azodiisobutyronitrile (AIBN) benzene, 80 °C, 18 h, 78%; (h) PdCl2, CuCl, O2, DMF-H2O (7:1), rt, 12 h, 90%; (i) NaOMe, MeOH, rt, 10 h, 70%. (j) TMSOTf, Et3N, THF, 0 °C, 0.5 h, then NBS, THF, 0 °C, 1 h, 80%. Figure 7: Formal total synthesis of the cortistatins. ( a ) 2,2-Dimethylpropane-1,3-diol, Pyridinium p-Toluenesulfonate (PPTS) benzene, 50 °C, 4 h, 80%; ( b ) KH, MeI, THF, 0 °C to room temperature (rt), 92%; ( c ) CAN, borate buffer (pH=8.0), 60 °C, 5 h, 55%; ( d ) ethynylmagnesium chloride, THF, 0 °C to rt, 75%+20% diastereomer; ( e ) NBS, AgNO 3 , acetone, rt, 0.5 h, 90%; ( f ) Ph 3 PAuNTf 2 (2.5 mol%), DCM, rt, 1 h, 81%; ( g ) allyl(Bu) 3 Sn, azodiisobutyronitrile (AIBN) benzene, 80 °C, 18 h, 78%; ( h ) PdCl 2 , CuCl, O 2 , DMF-H 2 O (7:1), rt, 12 h, 90%; ( i ) NaOMe, MeOH, rt, 10 h, 70%. ( j ) TMSOTf, Et 3 N, THF, 0 °C, 0.5 h, then NBS, THF, 0 °C, 1 h, 80%. Full size image To prepare intermediate 20 , ketone 23 was reacted with ethynylmagnesium chloride in THF at 0 °C to afford desired product 24 in 75% yield, together with its diastereisomer in 20% yield. The diastereoselective formation of product 24 could be a result of the chair-like transition state adopted by 23 , which might guide the nucleophile approaching from the bottom face of the ketone to achieve the minimum level of steric interaction (see three-dimensional structure of 23 in Fig. 7 ). Thus, bromination of the alkyne moiety in 24 with N -bromosuccinimide (NBS) in the presence of AgNO 3 in acetone at room temperature gave 20 in 90% yield. Treatment of substrate 20 with Ph 3 PAuNTf 2 (2.5 mol%) in DCM at room temperature for 1 h, gave desired product 19 in 81% yield. The structure of 19 was confirmed by X-ray crystallography of its derivative (see Supplementary Fig. 69 ). Product 19 was subjected to a radical-type allylation by reacting it with allyltributyl stannane in the presence of azodiisobutyronitrile (AIBN) and the resultant terminal alkene was then oxidized to diketone 25 via the Wacker oxidation to give diketone 25 in 70% yield over two steps. Thus, further treatment of diketone 25 with NaOMe in MeOH to initiate a cascade aldol condensation/β-elimination [69] , followed by an α-bromination with NBS in THF at 0 °C afforded 18 in 56% yield over two steps [70] . This compound has been used by Myers and colleagues [65] in the total synthesis of corstatins A , L , J and K . In summary, a novel strategy for the diastereoselective synthesis of structurally diverse oxabicyclo[3.2.1]octane scaffolds has been achieved via a gold-catalysed cascade reaction, which is consisted of three individual reactions, featuring (1) a gold-catalysed intramolecular nucleophilic addition of the OH group onto the carbon–carbon triple bond; (2) a gold-catalysed isomerization of exo-cyclic enol ether to a highly strained oxonium ion; (3) the oxonium-induced semi-pinacol rearrangement. This chemistry has also been demonstrated in the formal total synthesis of the cortistatins. DFT calculations reveal the necessity for the selective 1,2-alkyl migration to form oxabicyclo[3.2.1]octane scaffolds. Further applications of this methodology to other biologically active natural products with the oxabicyclo[3.2.1]heptane scaffold are currently underway in our laboratory. Materials For 1 H and 13 C NMR spectra of the compounds in this article, see Supplementary Figs 1–67 . For ORTEP diagrams, see Supplementary Figs 68 and 69 . General All reactions were conducted in oven-dried glassware under an inert atmosphere of dry nitrogen. All reagents were purchased and used without further purification unless otherwise specified. Solvents for flash column chromatography were technical grade and distilled before use. Analytical thin-layer chromatography was performed using silica gel plates with HSGF 254 (0.15–0.2 mm) manufactured by Shandong Huanghai Chemical Company (Qingdao, China). Visualization was performed by measuring ultraviolet absorbance (254 nm) and using the appropriate stain. Flash column chromatography was performed using Qingdao Haiyang Chemical HG/T2354-92 silica gel (45–75 mm). 1 H and 13 C NMR data were recorded on a Bruker 500 MHz (125 MHz for 13 C NMR) or a Bruker 400 MHz (100 MHz for 13 C NMR) nuclear resonance spectrometer unless otherwise specified. Chemical shifts (δ) in p.p.m. are reported relative to the residual chloroform signal ( 1 H 7.26 p.p.m. and 13 C 77.16 p.p.m.). Multiplicities are described as follows: s (singlet), bs (broad singlet), d (doublet), t (triplet), q (quartet) and m (multiplet). Coupling constants ( J ) are reported in Hertz (Hz). 13 C NMR spectra were recorded with total proton decoupling. High-resolution mass spectrometry electrospray ionization analysis was performed by the Analytical Instrumentation Center at Peking University, and High-resolution mass spectrometry data are reported as ion mass/charge ( m/z ) ratios in atomic mass units. General procedure for the gold-catalysed cascade reactions A mixture of Ph 3 PAuNTf 2 (2.5 mg, 0.005 mmol, 0.025 equiv) and AgNTf 2 (1.9 mg, 0.005 mmol, 0.025 equiv) in DCM (1.0 ml) was stirred for 0.5 h to generate the active gold catalyst in situ . The mixture was then added to a stirred solution of the substrate (0.20 mmol, 1.0 equiv) in DCM (4.0 ml) and stirred at ambient temperature for 2 h. The solvent was removed in vacuo , and the residue was purified by flash chromatography on silica gel to provide the desired product. For additional procedures see Supplementary Methods . Accession codes. The X-ray crystallographic coordinates for the structures reported in this article have been deposited at the Cambridge Crystallographic Data Centre (CCDC), under deposition number CCDC 1059110 (for S10 ) and 1059111 (for 12k ). These data can be obtained free of charge from the Cambridge Crystallographic Data Centre via http://www.ccdc.cam.ac.uk/data_request/cif . How to cite this article: Fu, J. et al. Towards a general diastereoselective route to oxabicyclo[3.2.1]octanes via a gold-catalysed cascade reaction. Nat. Commun. 6:8617 doi: 10.1038/ncomms9617 (2015).